The genome ofPrunus mume Prunus mume (mei), which was domesticated in China more than 3,000 years ago as ornamental plant and fruit, is one of the first genomes among Prunus subfamilies of Rosaceae been sequenced. Here, we assemble a 280M genome by combining 101-fold next-generation sequencing and optical mapping data. We further anchor 83.9% of scaffolds to eight chromosomes with genetic map constructed by restriction-site-associated DNA sequencing. Combining P. mume genome with available data, we succeed in reconstructing nine ancestral chromosomes of Rosaceae family, as well as depicting chromosome fusion, fission and duplication history in three major subfamilies. We sequence the transcriptome of various tissues and perform genome-wide analysis to reveal the characteristics of P. mume , including its regulation of early blooming in endodormancy, immune response against bacterial infection and biosynthesis of flower scent. The P. mume genome sequence adds to our understanding of Rosaceae evolution and provides important data for improvement of fruit trees. Rosaceae, with over 100 genera and 3,000 species, is the third most economically important plant family in temperate regions [1] . The Rosaceae family has been traditionally divided into four subfamilies according to fruit type: Rosoideae (Rosa, Fragaria, Potentilla and Rubus; fruit, achene; x =7, 8 or 9), Prunoideae (Prunus; fruit, drupe; x =8), Spiraeoideae (Spiraea; fruit, follicle or capsule; x =9) and Maloideae (Malus, Pyrus and Cotoneaster; fruit, pome; x =17) [2] . The poor phylogenetic resolution of the backbone of the Rosaceae phylogenetic tree suggests rapid evolutionary radiation of lineages within the family, corresponding to a relatively recent divergence of genera [3] . Possibly owing to this rapid evolution, Rosaceae members show significant phenotypic diversity, wherein common morphological synapomorphies are not readily identifiable. Plant habit, chromosome number and fruit type evolved independently within the family [2] , [3] , [4] . Rosaceous fruits are consumed in multiple forms, including fresh, dried, juice and processed products [5] . The economic importance of edible rosaceous crops is attributed to their flavourful fruits and nuts, which provide unique dietary contributions to consumers. Several Rosaceae species, including Malus × domestica (apple, 2 n =2 × =34) [6] , Fragaria vesca (strawberry, 2 n =2 × =14) [7] and Prunus persica (peach, 2 n =2 × =16) have already been sequenced. The P. mume (mei, 2 n =2 × =16) [8] is a woody perennial tree with a long intergeneration period of 3–5 years [9] . As the most famous ornamental flower and fruit tree in East Asian countries, P. mume has been domesticated for more than 3,000 years [9] . In East Asia, P. mume ’s flower and young fruit can tolerate low temperatures (−4 to −2 °C) in early spring [9] . P. mume blooms in late winter or early spring (typically late January or February) before the new leaves grow. The P. mume genome can be used to understand the structure of Rosaceae genomes in general and the rapid evolution of the Rosaceae genus. It will also help to measure and characterize the genetic diversity in domesticated and wild populations of fruit trees and determine how this diversity relates to the tremendous phenotypic diversity in fruit trees. Furthermore, genome-based tools can be developed to improve breeding work. Here, using the P. mume genomic sequence and the available M. × domestica and F. vesca genomic data, we reconstructed the ancestral genome of Rosaceae and analysed the evolution of the three chief genera Prunus, Malus and Fragaria. Our results were consistent with previous studies suggesting that small inversions had a significant function in the evolution of Rosaceae [10] . We identified 1,154 candidate genes that are critical to valuable traits, including flowering scent, flowering time and disease resistance. These genes, with the P. mume population material and the genetic markers that we developed, will be valuable for P. mume breeding and other Rosaceae species studies. Sequencing and assembly Constructing the reference genome for fruit trees is more challenging compared with other plants. The high heterozygosity of fruit trees, caused by artificial grafting and asexual reproduction, imposes technical challenges for the assembly algorithms [6] . The relatively long generation time and difficulties with the population materials impede construction of the genetic map. Further, the rapid evolution in Rosaceae prevents building chromosome structures according to collinearity. In order to construct the reference genome of P. mume , we initially sequenced two domesticated P. mume samples ( Supplementary Table S1 and Supplementary Methods ) using the Illumina Genome Analyser (GA) II. Both samples had a high heterozygous rate, as estimated using K-mer statistics ( Supplementary Fig. S1a and S1b ), and the de novo assembly results by current next-generation sequencing (NGS) algorithms did not meet the reference quality standards (data not shown). We then considered wild samples, owing to their lack of artificial grafting and asexual reproduction. We collected wild samples of P. mume in Tongmai, Bomi county, Tibet, China (30°06′N, 95°05′E, Supplementary Fig. S2 ), which is the western end of the region from which domesticated P. mume originated [11] , [12] . In a previous study [9] , [11] , [12] , we determined that the origin of P. mume was confined to an area of ~0.7 km 2 and that the primary distribution area was <0.3 km 2 below an altitude of 2,230 m. Samples from this region were highly homozygous owing to generations of self-fertilization in a hermetic geographic environment. We chose one such wild sample to be sequenced, and its low heterozygosity was confirmed by sequencing and K-mer statistics ( Supplementary Fig. S1c ). We generated 50.4 Gb of sequencing data for this wild sample using the Illumina GA II, including three short-insert (180–800 bp) pair-end libraries and five large-insert (2–40 Kb) mate-pair libraries ( Supplementary Table S2 ). SOAP denovo [13] , a genome assembler algorithm that is based on de Bruijn graph, was used to assemble the P. mume genome. Based on K-mer statistics, the P. mume genome was estimated to be 280 Mb ( Supplementary Fig. S1c ). Approximately 84.6% (237 Mb) of its genome was assembled. 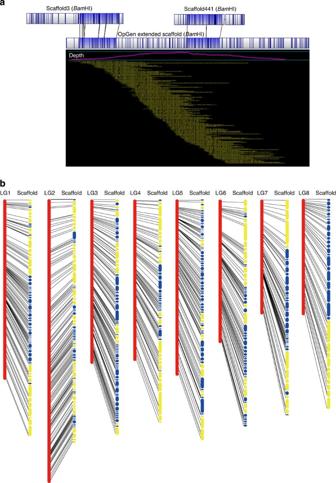Figure 1: WGM assembly and anchoring ofP. mumegenome. (a) Assembly ofP. mumegenome by WGM. (b) Anchoring theP. mumegenome into eight linkage groups using 779 high-quality SNP markers. Yellow scaffolds were anchored by WGM and SNP markers, whereas the blue scaffolds were anchored by SNP markers. The contig N50 of the assembled sequence was 31.8 Kb (longest, 201.1 Kb), and scaffold N50 was 577.8 Kb (longest, 2.87 Mb) ( Table 1 ). By mapping raw reads back to the draft genome, we observed a heterozygosity rate of 0.03% in this wild sample ( Supplementary Table S3 ), supporting our assumption of low heterozygosity in the wild sample. We identified 125,383 bp and 19,897 bp sequences in assembly similar to chloroplast and mitochondrial sequences, respectively ( Supplementary Table S4 ). Although most of the regions were shorter than 1,000 bp, we found a ~25,000 kb chloroplast-similar region, which might be the plasmid sequence or plastid-transferred nuclear fragment. Table 1 Statistics of P. mume genome assembly. Full size table To improve the assembly of the P. mume genome, we performed whole-genome mapping (WGM), an automated high-throughput optical mapping method [14] , to generate an entire genomic map ( Fig. 1a ). We constructed the WGM map with 300-fold whole-genome depth using BamHI and NheI independently. Through an iterative assembly strategy, combined with WGM and sequence data, 170 scaffolds that were assembled by NGS were grouped into 49 large scaffolds, thus the scaffold N50 improved significantly from 578 Kb to 1.1 Mb ( Table 1 ). Figure 1: WGM assembly and anchoring of P. mume genome. ( a ) Assembly of P. mume genome by WGM. ( b ) Anchoring the P. mume genome into eight linkage groups using 779 high-quality SNP markers. Yellow scaffolds were anchored by WGM and SNP markers, whereas the blue scaffolds were anchored by SNP markers. Full size image Then we constructed a high-density genetic map by applying restriction-site-associated DNA (RAD) marker strategy [15] in a segregating F 1 population. The consensus genetic map contained eight linkage groups, consisted of a set of 1,484 high-quality single-nucleotide polymorphism (SNP) markers (co-dominate markers), 779 of which were used in anchoring and orienting scaffolds ( Fig. 1b ). The genetic map improves the quality of the reference and will be useful in molecular marker-assisted breeding and further map-based cloning. Genome annotation We annotated 106.8 Mb (45.0% of the assembled genome) of repetitive sequences ( Supplementary Table S5 ) in the P. mume genome by integrating the de novo and homologue-based approaches. Transposable elements (TEs) were the predominant components, constituting 97.9% of all repetitive sequences. The long terminal repeat Copia family and Gypsy family were the most abundant TEs in the P. mume genome. The TE divergence rate suggested a lack of recent amplification ( Supplementary Fig. S3 ). These were conserved in M. × domestica and F. vesca while the M. × domestica have a much higher proportion in Gypsy family than P. mume and F. vesca ( Supplementary Table S6 ). To improve the gene annotation, we generated 11.3 Gb of RNA-Seq data from five major tissues: bud, fruit, leaf, root and stem ( Supplementary Table S7 ). Using these data, integrated with ab initio homologue prediction methods (Methods), we annotated 31,390 protein-coding genes, comparable with the value in F. vesca (34,809) [7] and less than in M. × domestica (57,386) [6] , as expected. The transcript length in P. mume was 2,514 bp on average, with 4.6 exons per gene ( Supplementary Table S8 ). Approximately 82.5% of all genes could be functionally annotated following a consensus method of either known homologous or predictive sequence signatures using Swissprot, GO, TrEMBL [16] , InterPro [17] or KEGG [18] . About 98.3% of these annotations were not hypothetical or uncharacterized, and we considered them as high confidence ( Supplementary Table S9 ). We noted that 25,854 (82.6%) gene models were expressed, of which 768, 308, 240, 762 and 179 genes were expressed solely in bud, fruit, leaf, root and stem, respectively. We further integrated 82,832 peach expressed sequence tag (EST) sequences, together with RNAseq data, 85.1% of gene models represented as transcripts. We also annotated the non-coding RNA genes in the current assembly including 508 transfer RNA, 209 microRNA, 125 ribosomal RNA and 287 small nuclear RNA ( Supplementary Table S10 ). Genome evolution By genome self-alignment by MCscan [19] ( Supplementary Fig. S4 , Method) and the number of transversions at fourfold degenerate sites (4DTv) distribution of duplicated pairs, there was no recent whole-genome duplication (WGD) after species differentiation between P. mume and M. × demestica ( Fig. 2a ). 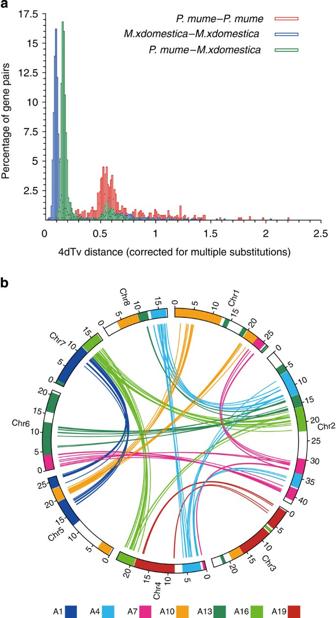Figure 2: The evolution ofP. mume. (a) 4DTv distribution of duplicate gene pairs inP. mumeandM.×domestica, calculated based on alignment of codons with the HKY (Hasegawa, Kishino and Yano) substitution model. (b) The duplication ofP. mumeby paralogous pairs in theP. mumegenome (chromosomes Chr1–Chr8). Each line represents a duplicated gene. The seven colours reflect the seven ancestral eudicot linkage groups (A1, A4, A7, A10, A13, A16 and A19). Figure 2: The evolution of P. mume . ( a ) 4DTv distribution of duplicate gene pairs in P. mume and M. × domestic a, calculated based on alignment of codons with the HKY (Hasegawa, Kishino and Yano) substitution model. ( b ) The duplication of P. mume by paralogous pairs in the P. mume genome (chromosomes Chr1–Chr8). Each line represents a duplicated gene. The seven colours reflect the seven ancestral eudicot linkage groups (A1, A4, A7, A10, A13, A16 and A19). Full size image We examined the paleo-history in Prunus and found that there was a triplicated arrangement (ancestral γ event). We aligned 27,819 gene models to the seven paleo-hexaploid ancestor chromosome groups in grape [20] and identified that the colinearity blocks contained 2,772 orthologs, the extent of these blocks covered 78.1% of the P. mume genome. Further, we aligned 27,819 P. mume gene models to themselves and identified seven major blocks of duplication, which corresponded to 194 gene pairs, covering 38.5% of the anchored genome. The chromosome-to-chromosome relationships P5–P7, P2–P4–P8, P1–P2–P4–P6, P1–P5, P2–P6–P8, P2–P4–P7 and P3–P4 ( Fig. 2b and Supplementary Table S11 ) suggested that triplicated arrangement (γ event) marks remained in the P. mume genome. Based on evidence of paleo-hexaploidization (γ event) and lineage-specific duplications in eudicots, it was possible to examine chromosomal changes during the evolution of P. mume and other Rosaceae species. Reconstruction of ancestral chromosomes of Rosaceae We reconstructed nine ancestral chromosomes of the Rosaceae family and determined the history of chromosome fusion, fission and duplication in the three major Rosaceae subfamilies. Previous studies have reported the eudicots ancestor with seven proto-chromosomes [20] and the grass ancestor with five proto-chromosomes [21] . Using M. × domestica as a reference, we analysed the syntenic relationships among the P. mume (P), F. vesca (F) and M. × domestica (M). One hundred and fifty-one blocks that contained 4,546 orthologous genes, covering 96.9% of the anchored P. mume genome, were identified between P. mume and M. × domestica versus 132 blocks with 2,031 orthologous genes, covering 88.8% of the F. vesca genome, between F. vesca and M. × domestica . The chromosome-to-chromosome orthologous relationships were shown in Supplementary Fig. S5 and Supplementary Table S12 . Combining the intergenomic and intragenomic analysis of the Rosaceae genomes, we noted the following primary chromosome pair combinations: M5–M10/P3–P6/F2–F3, M3–M11/P1–P3–P6/F2–F3–F5, M9–M17/P2–P4/F1–F6, M13–M16/P2/F4, M4–M12–M14/P1–P2–P6–P8/F5–F6, M6–M14/P7/F5, M1–M2–M7/P5/F7, M8–M15/P2/F2–F5 and M1–M2–M15/P1–P2–P3–P8/F1 ( Supplementary Fig. S5 ). We reconstructed a putative ancestral genome of Rosaceae and proposed an evolutionary scenario of P. mume , M. × domestica and F. vesca from the putative 9-chromosome ancestor ( Fig. 3 ). 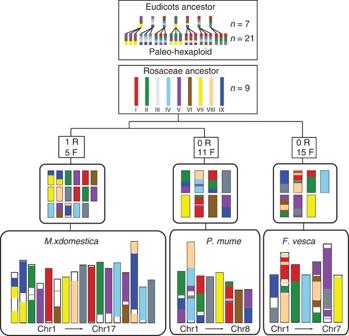Figure 3: Evolutionary model of Rosaceae genome. The Rosaceae ancestor chromosomes are represented by nine colours. The various evolutionary processes from the common ancestor are indicated as R (WGD) and F (fusions of chromosomes). In the second layer, different colours in each chromosome represent origin from the common ancestral chromosomes. The current structure of the Rosaceae genomes is shown at the bottom of the figure. In some regions, we were not able to determine which ancestral chromosome they came from, and those regions were represented as white spaces. Figure 3: Evolutionary model of Rosaceae genome. The Rosaceae ancestor chromosomes are represented by nine colours. The various evolutionary processes from the common ancestor are indicated as R (WGD) and F (fusions of chromosomes). In the second layer, different colours in each chromosome represent origin from the common ancestral chromosomes. The current structure of the Rosaceae genomes is shown at the bottom of the figure. In some regions, we were not able to determine which ancestral chromosome they came from, and those regions were represented as white spaces. Full size image In P. mume , chromosomes 4, 5 and 7 did not undergo rearrangement, coming directly from ancient chromosomes III, VII and VI, respectively. Chromosome 1 came from ancestral chromosome II, V and IX. Chromosome 2 originated from ancient chromosome IV and VIII into which some of chromosomes III and V were inserted. Chromosome 3 came from chromosomes I, II and IX; chromosome 6 came from I, II and V; and chromosome 8 originated from ancient chromosomes V and IX. Thus, we hypothesized that at least 11 fissions and 11 fusions occurred in P. mume from the nine common ancestral chromosomes. For M. × domestica , at least one WGD and five fusions took place to reach the 17-chromosome structure, compared with 15 fusions for F. vesca to effect the 7-chromosome structure. Early blooming of P. mume P. mume is one of the first trees that bloom in early spring, blooming even below 0 °C. Thus, P. mume has a system to acclimate to cold weather and release itself from dormancy. The dormancy-associated MADS-box transcription factors (DAM) family, which is related to dormancy induction and release [22] , was identified in the P. mume assembly, and all six DAM genes were noted in the tandem array ( Fig. 4a , Supplementary Table S13 ). Sasaki et al. [22] identified six DAM genes, all of which were transcriptional repressors in P. mume . They also found that all DAM genes were repressed during prolonged exposure to cold and maintained at low levels until endodormancy release. Jimenez [23] observed that the expression of DAM3, DAM5 and DAM6 was suppressed by cool temperatures, bottoming on bud break in P. persica . These findings suggest that the DAM genes inhibit dormancy release and their expression are suppressed during prolonged exposure to cold to allow bud release from dormancy. 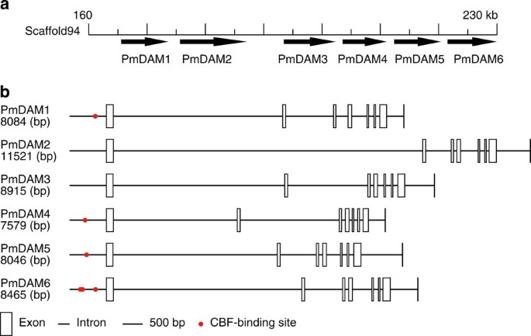Figure 4: Six tandemly arrayed DAM genes inP. mume. (a) Overview of PmDAM in theP. mumegenome. Six PmDAM genes are located as tandem repeats. (b) Structures of PmDAM genes inP. mume. Boxes and lines represent exons and introns, whereas red points represent CBF-binding site. Figure 4: Six tandemly arrayed DAM genes in P. mume . ( a ) Overview of PmDAM in the P. mume genome. Six PmDAM genes are located as tandem repeats. ( b ) Structures of PmDAM genes in P. mume . Boxes and lines represent exons and introns, whereas red points represent CBF-binding site. Full size image We hypothesized that the DAM genes explained the early dormancy release of P. mume . To this end, we examined the phylogenetic relationships among DAM genes in P. mume using the PHYML 3.0 software. The molecular evolution models of the six tandem DAM genes in P. mume suggested that they were derived from serial duplication events in the following order: PmDAM1, PmDAM3, PmDAM2, PmDAM5, PmDAM4 and PmDAM6 ( Supplementary Fig. S6 ). This model was consistent with previous studies in the peach genome [24] , and we suggest that these duplication events are unique in the Prunus subfamily—we did not find these tandem DAM genes in M. × domestica or F. vesca . Two other programs, MEGA 4 (ref. 25 ) and PAML4 (ref. 26 ), obtained similar results. By estimation of pairwise dN and dS rates using MEGA 4, there was significant purifying selection and no significant positive selection of the six sequences. In an analysis of P. mume DAM genes, most sites were highly conserved, with a dN/dS rate ratio near 0, or nearly neutral. In addition to DAM, C-repeat-binding transcription factors (CBF) mediate the establishment of early dormancy release—overexpression of PpCBF1 in M. × domestica results in strong sensitivity to short day lengths and induced dormancy at optimal growth temperatures [27] . Horvath et al. [28] noted that EeDAM1 was cold stress-responsive and contained putative CBF-binding sites, which were cis -regulating motifs that were targeted by the cold/drought stress CBF regulon in the 2,000-bp region upstream of the EeDAM1 translation start codon. This finding suggests that CBF control the cold-responsive EeDAM1 gene [28] . Similar to EeDAM1, conserved CBF sites were identified in the 1,000-bp region upstream of the translation start codons in DAM4–DAM6 in peach and Japanese apricot [22] , [24] . In the P. mume genome, we identified 13 CBF orthologous genes ( Supplementary Table S14 ) and 7 CBF regulons, late embryogenesis-abundant proteins/dehydrins [29] ( Supplementary Table S15 ). In the upstream regions of DAM genes in P. mume , we noted more putative CBF-binding sites on DAM4, DAM5 and DAM6 than in peach, and found novel sites, one on DAM1 and two on DAM6 ( Fig. 4b ). We suggest that these additional sites render P. mume more sensitive to cold and result in early blooming in spring. In summary, our analyses have increased our understanding of the molecular control of dormancy, flowering regulation and acclimation to cold. The CBF and DAM genes that we identified in P. mume might allow molecular biology facilities to breed ornamental plants and fruits with disparate blooming times. Disease resistance-related genes and pathogenic interaction The search for natural disease resistance is a chief objective in P. mume breeding. In the P. mume genome, we identified 253 leucine-rich repeat receptor-like kinase (LRR-RLK) genes, comparable with the number in Arabidopsis thaliana [30] (221) and Theobroma cacao [31] (253) and less than in Populus trichocarpa [32] (436) ( Supplementary Table S16 ). The LRR-XI and LRR-XII subfamilies expanded tremendously in the P. mume genome compared with Arabidopsis thaliana [30] ( Supplementary Table S17 ); similar expansions have been observed in T. cacao [31] and P. trichocarpa [32] . The nucleotide-binding site-coding resistant gene (NBS-coding R gene) is one of the largest families in P. mume , with 411 members, more than twice that of A. thaliana [33] and F. vesca [7] ( Supplementary Table S18 ). Pathogenesis-related (PR) proteins are plant-coded proteins are induced by various stress stimuli. PR proteins mediate plant defence against pathogenic constraints and general adaptation to stressful environments [34] . Most PR gene families in P. mume were expanded notably and were arranged in tandem, especially PR10 (22 of 25) ( Supplementary Table S19 ). By genomic analysis, the majority of PR10 members in P. mume formed a cluster of <100 Kb ( Supplementary Table S20 , Supplementary Fig. S7 ), but we did not find this cluster in the other sequenced Rosacea genomes. Further, the PR10 families encode hypothetical proteins that are highly expressed at the transcriptional level in roots and leaves in P. mume ( Supplementary Fig. S8 ). Thus, the expansion of the PR10 family might be related to the response of P. mume to salt, drought and fungal infection in the roots and leaves [35] , [36] , [37] . Floral scent Floral scent, determined by a complex mixture of low-molecular-weight volatile molecules, has significant function in the reproductive processes of many plants and enhances the aesthetic properties of ornamental plants [38] . In earlier research, we determined that the dominant compound classes in P. mume flowers were benzenoid/phenylpropanoid from the cinnamic acid pathway and that terpene compounds were also present. Genes related to the biosynthesis of volatile compounds, such as benzyl alcohol acetyltransferase (BEAT), which catalyses the synthesis of benzyl acetate [39] , were identified in the P. mume genome. The BEAT gene family expanded notably in P. mume (34 members) compared with Malus × domestics (16), F. vesca (14), Vitis vinifera (4), P. trichocarpa (17) and A. thaliana (3) ( Supplementary Table S21 ). Twenty-six of 34 P. mume BEAT genes lay in clusters, the largest of which contained 12 members that were arranged in tandem ( Supplementary Fig. S9 , Supplementary Table S22 ), suggesting that BEAT genes originated from serial duplication events, unlike the other sequenced plants. In summary, the expansion of the BEAT gene family might increase the content of benzyl acetate and be related to the special fragrance of P. mume. Research on the P. mume genome should allow us to breed novel aromatic cultivars and other aromatic plants in the Rosaceae family. We are eager to establish an appropriate reference genome in Rosids species, which includes one-third of all flowering plants [40] . Currently, draft genome sequences are available for genome-level comparisons and analysis in three model Rosaceae species— M. × domestica , F. vesca and P. mume . The domesticated apple ( M. × domestica ), the main fruit crop of temperate regions throughout the world, is highly heterozygous and has a large genome, which creates technical challenges in assembling its genome, resulting in 1,629 metacontigs. The strawberry ( F. vesca ) has a much smaller genome of ~240 Mb, allowing functional gene studies within Rosaceae. Although the strawberry is useful for functional genomics research, most related high-value fruit plants in the Rosaceae species—peach ( P. persica ), pear ( Pyrus nivalis ) and cherry ( Prunus avium )—are woody plants, not herbaceous. Unfortunately, the nearest relatives of woody fruit crops usually have a cumbersome polyploid genome. After a detailed study of its origin and the current distribution in P. mume , we obtained a suitable sample from an isolated group in the area origin of P. mume for genomic sequencing and assembly. We successfully assembled the genomic sequence of P. mume by NGS data owing to its small genome of ~280 Mb and low heterozygosity. With WGM, we increased the scaffold quality to 1.1 Mb in N50 and constructed P. mume pseudochromosomes using 779 SNP markers from eight linkage groups. We conclude that the combination of Illumina GA, WGM technologies and the genetic map constructed by RAD can be used to perform de novo sequencing of plant genomes, allowing high-quality, rapid and low-cost sequencing of other plant species with similar genomic composition. The sequence of the P. mume genome is a valuable resource for biological research and breeding. Based on the sequences of P. mume , M. × domestica and F. vesca , we reconstructed nine ancestral chromosomes of the Rosaceae family and inferred that they were shaped from an ancestor. The genome also increases our knowledge of the evolution of the Rosaceae. The analysis of the P. mume genome and transcriptome can provide insights into the mechanisms of flowering scent, flowering dormancy and disease resistance. Note added in proof : A paper describing in detail the full protocols used for the optical whole genome mapping has recently been published [52] . DNA preparation and whole-genome shotgun sequencing We used a whole-genome shotgun sequencing strategy with the Illumina GA. Total DNA was extracted from fresh young leaves of the wild species in Tongmai town, Tibet, China (accession No. BJFU1210120008), with the plant genomic DNA extraction Kit (Tiangen, Beijing, China) following the manufacturer’s instructions. To obtain enough DNA to construct and sequence the library, we performed whole-genome amplification. We constructed eight paired-end sequencing libraries with insert sizes of ~180, 500, 800 bp, 2, 5, 10, 20 and 40 kb. For small-insert libraries, 5 μg of DNA were sheared to fragments of 180–800 bp, end-repaired, A-tailed and ligated to Illumina paired-end adapters (Illumina). The ligated fragments were size selected at 180, 500 and 800 bp on agarose gel and amplified by ligation-mediated PCR to produce the corresponding short-insert libraries. For long-insert size library construction, 20–40 μg of genomic DNA were sheared to the desired insert size using nebulization for 2 kb or HydroShear (Covaris) for 5, 10, 20 and 40 kb. Next, the DNA fragments were end-repaired using biotinylated nucleotide analogues, size selected at 2, 5, 10, 20 and 40 kb and circularized by intramolecular ligation. Circular DNA molecules were sheared with Adaptive Focused Acoustic (Covaris) to an average size of 500 bp. Biotinylated fragments were purified with magnetic beads (Invitrogen, CA, USA), end-repaired, A-tailed and ligated to Illumina paired-end adapters, size-selected again and purified by ligation-mediated PCR. In total, we generated 50.4 Gb data of paired ends (PEs), ranging from 50 to 100 bp. These data were checked and filtered on the reads that were generated [13] . We filtered the low-quality reads with following filtering criteria: reads had an ‘N’ over 10% of their length; reads contained more than 40-bp low-quality bases (quality score ≤5); reads contained more than 10-bp adapter sequences (allowing ≤2 bp mismatches); small-insert size paired-end reads that were overlapped (≥10 bp); and Read1 and Read2 of paired-end reads were completely identical that meant these paired-end reads were determined to be artefacts of PCR experiment. Using stringent criteria, 28.4-Gb high-quality data were used for de novo genome assembly. Genome assembly We performed whole-genome assembly using SOAP denovo (Version 1.05) [13] with high-quality reads. SOAP denovo loaded reads into computer memory and constructed de Bruijn graph. The graph was simplified, broke the connections at repeat boundaries and output the unambiguous sequence fragments as contigs. After realigned all usable reads to the contig sequences and obtained aligned PEs, SOAPdenove calculated the number of shared PEs relationships between each pair of contigs, weighed the rate of consistent and conflicting PEs, and constructed the scaffolds step by step. To close the gaps inside the constructed scaffolds, which were composed primarily of repeats that were masked before scaffold construction, we used the PEs information to retrieve the read pairs that had one end mapped to the unique contig and the other located in the gap regions and performed local assembly using GapCloser (v1.12, http://soap.genomics.org.cn/down/GapCloser_release_2011.tar.gz ) with these collected reads. Whole-genome mapping High-quality DNA (high molecular weight, >200 kb) that was specific for WGM was prepared from fresh P. mume leaves. Whole-genome shotgun single-molecule restriction maps were generated with the automated Argus system (OpGen Inc., MD, USA). First, DNA molecules were deposited onto silane-derivatized glass surfaces in MapCards (OpGen Inc.) and digested with Nhe I or Bam HI for 20 min. Then, the DNA was stained with JOJO fluorescent dye (Invitrogen) and imaged with the Argus system. Overall, 243,174 single-molecule restriction maps (>250 kb) with an average size of 344 kb were generated. The total size was ~83.6 Gb. When using WGM data to extend scaffolds, the original scaffold sequences were first digested in silico to generate corresponding restriction maps for each scaffold. Then, the in silico restriction maps were used as seeds to identify single molecules by length-based alignment using the Genome-Builder TM software package ( http://www.opgen.com/products-and-services/softwares/genome-builder ). These single-molecule maps were assembled together to extend the scaffolds with consensus restriction maps. Meanwhile, the scaffolds with low-coverage regions at both ends were trimmed, and only the high-quality extensions remained. To extend sufficient scaffolds, this alignment–assembly process was iterated four times. All pairwise alignments were considered initial candidates for scaffold connection. The alignments with the highest scores remained when conflicts occurred. Super-scaffolds were constructed using the adjacent overlapping relationships between scaffolds; simultaneously, the orientation between each pair of scaffolds could be determined. The details on scaffold alignment and orientation can be obtained from the manufacturer of OpGen. Genetic map construction and scaffold anchoring A total of 260 F 1 seedlings of the cross between ‘Fenban’ and ‘Kouzi Yudie’ were used to construct the linkage map. The linkage analysis was performed using JoinMap, version 3.0 (ref. 41 ). RAD-based SNP markers were first tested against the expected segregation ratio. Two heterozygous SNP alleles between two parents were expected to segregate at a 1:2:1 ratio. One heterozygous and one homozygous SNP allele between two parents were expected to segregate at a 1:1 ratio. Distorted markers ( P <0.01) were filtered to construct a genetic map by χ 2 test. Then, reads that contained SNP markers were aligned to the scaffolds. Only unique aligned SNPs with a cutoff of 87.5% identity remained, per BLAT [42] (coverage ≥0.90). An LOD score of 12.0 was initially set as the linkage threshold for linkage group identification. Eight linkage groups that had the same number of P. mume chromosomes were formed at an LOD threshold of 12.0. All SNP markers were used to construct the P. mume consensus map with the CP population model in JoinMap, version 3.0. To reduce the complex of scaffolds that were anchored to hundreds of SNP markers, a tag SNP was selected from each scaffold with multiple SNPs. We calculated the recombination fractions between all pairs of SNPs in a scaffold and chose the SNP that had the minimum recombination fraction in the sum. Tag SNPs were used to identify the order of scaffolds. Then, two marginal SNPs were used to orient the scaffolds. Scaffolds with only one SNP marker could be anchored but not oriented owing to a lack of markers. One hundred scaffolds (18% of 567 scaffolds) were labelled ‘uncertain orientation.’ Gene prediction To predict genes, four approaches were used: de novo prediction, homology-based method, EST-based method and transcript-to-genome sequences. For de novo prediction, Augustus [43] , GENSCAN [44] and GlimmerHMM [45] were used with parameters trained on A. thaliana . For the homology search, we mapped the protein sequences of four sequenced plants ( Cucumis sativus , Carica papaya , F. vesca and A. thaliana ) onto the P. mume genome using TBLASTN, with an E-value cutoff of 1e-5, and homologous genomic sequences were aligned against matching proteins using GeneWise [46] for accurate spliced alignments. In the EST-based prediction, 4,699 ESTs of P. mume were aligned against the P. mume genome using BLAT [42] (identity ≥0.95 and coverage ≥0.90) to generate spliced alignments. The de novo set (28,610 to 36,095), four homologue-based results (24,277 to 29,586) and EST-based gene set (2001) were combined by GLEAN [47] to integrate a consensus gene set. Short genes (CDS length <150 bp) and low-quality genes (gaps in more than 10% of the coding region) were filtered. To finalize the gene set, we aligned RNA-Seq data from bud, fruit, leaf, root and stem to the genome using Tophat [48] (Version 1.2.0, implemented with bowtie1 Version 0.12.5), and the alignments were used as input for Cufflinks [49] (Version 0.93) with default parameters. Open reading frames of those transcripts were predicted using structure parameters trained on perfect genes from homology-based prediction. In the end, based on their coordinates on the genome sequences, we manually combined the Glean gene set and open reading frames of transcripts to form the final gene set that contains 31,390 genes. Comparative genome analyses Paralogues and orthologues genes were identified by BLASTP search (E-value cutoff of 1e-5). After removing self-matches, syntenic blocks (≥5 genes per block) were identified, based on MCscan [19] . The aligned results were used to generate dot plots—for self-aligned results, each block represents the paralogues region that arose from genome duplication, and for inter-aligned results, each block represents the orthologous region that was derived from a common ancestor. We calculated 4DTv for each gene pair in the block and drew the distribution of 4DTv values to estimate the speciation between species or WGD events. Identification of duplicate and syntenic regions Three new parameters, defined in Salse et al. [50] , were used to identify paralogous and orthologous relationships between P. mume , M. × domestica , F. ve sca and V. vinifera by BLASTN. Paralogous gene pairs that were identified during duplication analysis in P. mume and M. × domestica, respectively, and orthologous gene pairs that were identified by colinearity analysis between P. mume and M. × domestica , F. ve sca and M. × domestica , and P. mume and V. vinifera were validated by CloseUp [51] analysis. Based on the syntenic and duplicate relationships, Rosaceae ancestral chromosomes were reconstructed, and the paleo-history was analysed. How to cite this article: Zhang, Q. et al. The genome of Prunus mume . Nat. Commun. 3:1318 doi: 10.1038/ncomms.2290 (2012). Accession codes: P. mume genome sequencing data have been deposited at NCBI BioProject under accession PRJNA171605. Sequencing data for P. mume and RAD analyses are available in the NCBI Sequence Read Archive (SRA) under accessions SRA056478 and SRA057102 . P. mume RNAseq data are available in the NCBI Gene Expression Omnibus (GEO) under accessions GSE40162 . Full assembly and analysis data are available at http://prunusmumegenome.bjfu.edu.cn .